Common variants in Alzheimer’s disease and risk stratification by polygenic risk scores Genetic discoveries of Alzheimer’s disease are the drivers of our understanding, and together with polygenetic risk stratification can contribute towards planning of feasible and efficient preventive and curative clinical trials. We first perform a large genetic association study by merging all available case-control datasets and by-proxy study results (discovery n = 409,435 and validation size n = 58,190). Here, we add six variants associated with Alzheimer’s disease risk (near APP, CHRNE, PRKD3/NDUFAF7, PLCG2 and two exonic variants in the SHARPIN gene). Assessment of the polygenic risk score and stratifying by APOE reveal a 4 to 5.5 years difference in median age at onset of Alzheimer’s disease patients in APOE ɛ4 carriers. Because of this study, the underlying mechanisms of APP can be studied to refine the amyloid cascade and the polygenic risk score provides a tool to select individuals at high risk of Alzheimer’s disease. Thus far, multiple loci associated with Alzheimer’s disease (AD) have been described next to causal mutations in two subunits of γ-secretases, membrane-embedded aspartyl complexes ( PSEN1 , PSEN2 genes ) , and the gene encoding one target protein of these proteases, the amyloid precursor protein gene (APP) . The most prominent locus, APOE , was detected almost 30 years ago using linkage techniques [1] . In addition, genome-wide association studies (GWAS) of AD case-control datasets and by-proxy AD case-control studies have identified 30 genomic loci that modify the risk of AD [2] , [3] , [4] , [5] , [6] , [7] . These signals account for ~31% of the genetic variance of AD, leaving most of the genetic risk as yet uncharacterized [8] . Further disentangling the genetic constellation of common genetic variations underlying AD can drive our biological insights of AD and can point toward novel drug targets. There are over 50 million people living with dementia and the global cost of dementia is well above 1 trillion US$ [9] . This means there is a medical and economical urgency to efficiently test interventions that are under development. Therefore, to increase power and reduce duration of trials, pre-symptomatic patients that are at high genetic risk of disease are increasingly developed [10] . However, only carriers of causal mutations ( APP, PSEN1, and PSEN2 ) and the APOE ɛ4 allele are considered high risk, while other common and rare genetic variants are ignored [11] . Despite that, the combined effects of all currently known variants in a polygenic risk score (PRS) is associated with the conversion of mild cognitive impairment to AD [12] , [13] , the neuropathological hallmarks of AD, age at onset (AAO) of disease [14] , [15] , [16] , [17] and lifetime risk of AD [18] . In this work we aim to comprehend and expand the knowledge of the genetic landscape underlying AD and provide additional evidence that a PRS of variants can be a robust tool to select high risk individuals with an earlier AAO. We first performed a meta-GWAS integrating all currently published GWAS case-control data, by-proxy case-control data, and the data from the Genome Research at Fundació ACE (GR@ACE) study [19] . We confirm the observed associations in a large independent replication study. Then, we construct an update of the PRS and test whether the effects of the PRS are influenced by diagnostic certainty, sex and AAO groups. Lastly, we test whether the PRS could be used to identify individuals at the highest odds of having AD and we compared AAO of the AD cases. This study describes the identification of six variants associated with AD risk and provides an extended PRS tool to select individuals at high risk of AD. Meta-GWAS of AD We combined data from three AD GWASs: the summary statistics calculated from the GR@ACE [19] case-control study (6331 AD cases and 6055 controls), the IGAP [20] case-control study (up to 30,344 AD cases and 52,427 controls) and the UKB AD-by-proxy case-control study [21] (27,696 cases of maternal AD with 260,980 controls, and 14,338 cases of paternal AD with 245,941 controls, Fig. 1 , Supplementary Data 1 ). Although we observed inflation in the resulting summary statistics ( λ median = 1.08; see Supplementary Fig. 1d ), it was not driven by an un-modeled population structure (LD score regression intercept = 1.036). The full details of the studies are described in methods. After study-specific variant filtering and quality-control procedures, we performed a fixed effects inverse-variance-weighted meta-analysis [22] on the summary statistics of the three studies. Using this strategy, we identified a genome-wide significant (GWS) association ( p < 5 × 10 −8 ) for 36 independent genetic variants in 35 genomic regions (the APOE region contains signals for ɛ4 and ɛ2). As a sensitivity analysis, we removed the AD-by-proxy study and compared the resulted effect estimates with and without this dataset. We found a high correlation between the effect estimates from the case-control and by-proxy approaches for the significant loci ( R 2 = 0.994, p = 8.1 × 10 −37 ; Supplementary Fig. 1e ). Four genomic regions were not previously associated with AD (see Manhattan Plot, Fig. 2a ). Fig. 1: Flow chart of analysis steps. Discovery meta-analysis in GR@ACE, IGAP stage 1 + 2 and UKBiobank followed by a replication in 16 independent cohorts. The genome-wide significant signals found in meta-GWAS were used to perform a Polygenic Risk Score in a clinical and pathological AD dataset. See Supplementary Methods to more information about the cohorts included and methods to the PRS generation. a Extended dataset (Moreno-Grau et al. [19] ), b StageI + StageII (Kunkle et al. [20] ), c By proxy AD: Meta-analysis of maternal and paternal history of dementia (Marioni et al. [21] ), d Extra and independent GR@ACE dataset incorporated only for replication purposes, e Pathologically confirmed AD cases, f AD cases diagnosed based on clinical criteria, g Controls participants aged 55 years and younger. N = Total of individuals within specified data. Full size image Fig. 2: GWAS meta-analysis for AD risk ( N = 467,623). a Manhattan plot of overall meta-analysis for genome-wide association in Alzheimer’s disease highlighting in pink the loci associated with AD in this study ( PRKD3/NDUFAF7, SHARPIN, CHRNE, PLCG2 , and APP ). b – f Locus plots for the signals associated with AD in overall meta-analysis results. Full size image Next, we aimed at replicating the associated loci in 16 cohorts (19,087 AD cases and 39,101 controls in total), many of them collected and analyzed by the European Alzheimer’s Disease Biobank (JPND-EADB) project. We tested all variants with suggestive association ( p < 10 −5 ) located within a 200 kb region from the sentinel SNP. Overall, 384 variants were tested in the replication datasets (Supplementary Data 2 ). 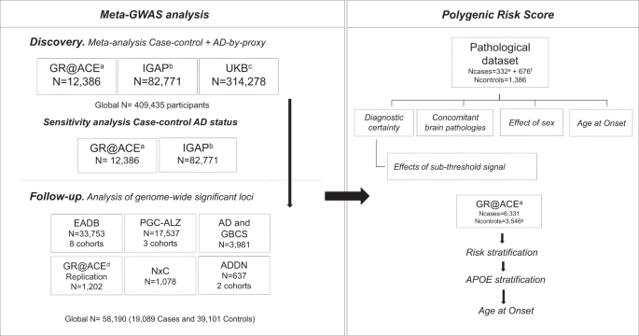Fig. 1: Flow chart of analysis steps. Discovery meta-analysis in GR@ACE, IGAP stage 1 + 2 and UKBiobank followed by a replication in 16 independent cohorts. The genome-wide significant signals found in meta-GWAS were used to perform a Polygenic Risk Score in a clinical and pathological AD dataset. SeeSupplementary Methodsto more information about the cohorts included and methods to the PRS generation.aExtended dataset (Moreno-Grau et al.19),bStageI + StageII (Kunkle et al.20),cBy proxy AD: Meta-analysis of maternal and paternal history of dementia (Marioni et al.21),dExtra and independent GR@ACE dataset incorporated only for replication purposes,ePathologically confirmed AD cases,fAD cases diagnosed based on clinical criteria,gControls participants aged 55 years and younger.N= Total of individuals within specified data. Discovery and replication were combined, and we identified associations in six variants comprising five genomic loci annotated using FUMA [23] (Table 1 , Fig. 2b–f , Supplementary Fig. 2 and Supplementary Results ). In APP , we identified a common (MAF = 0.46) intronic variant associated with a reduced risk of AD (rs2154481, OR = 0.95 [0.94–0.96], p = 1.39 × 10 −11 , Fig. 2f ). In SHARPIN (SHANK Associated RH Domain Interactor) gene, we found two missense mutations (rs34173062/p.Ser17Phe and rs34674752/p.Pro294Ser) that are in linkage equilibrium ( R 2 = 1.3 × 10 −6 , D ′ = 0.014, p = 0.96). Both missense variants increased AD risk (p.Ser17Phe, MAF = 0.085, OR = 1.14 [1.10–1.18], p = 9.6 × 10 −13 and p.Pro294Ser, MAF = 0.052, OR = 1.13 [1.09–1.18], p = 1.0 × 10 −9 , Fig. 2b ). A variant close to the genes PRKD3 and NDUFAF7 (rs876461, MAF = 0.143) emerged as the most significant variant in the region after the combined analysis (OR = 1.07 [1.05–1.09], p = 1.3 × 10 −9 , Fig. 2c ). In the 3’-UTR region of CHRNE (Cholinergic Receptor Nicotinic Epsilon Subunit), rs72835061 (MAF = 0.085) was associated with a 1.09-fold increased risk of AD (95% CI [1.06–1.11], p = 1.5 × 10 −10 , Fig. 2e ). Our analysis also strengthened the evidence of association with AD for three additional genomic loci including an association with a variant in PLCG2 (rs3935877, MAF = 0.13, OR = 0.92 [0.90–0.95], p = 6.9 × 10 −9 , Fig. 2d ), and confirmed another common variant in PLCG2 , a stop gain mutation in IL-34 and a variant near HS3ST1 (Table 1 , Supplementary Fig. 3 and Supplementary Data 2 , 3 ). We were not able to replicate two loci ( ELK2AP and SPPL2A regions) that showed suggestive association with AD ( p < 1 × 10 −7 in discovery). Table 1 Association for the AD loci selected for follow-up. Full size table Polygenic risk scores In order to assess the robustness and combined effect of the genetic landscape of AD (Fig. 3 , Supplementary Data 4 ), we constructed a weighted PRS based on the 39 genetic variants (excluding APOE genotypes) that showed GWS evidence of association with AD (see Methods, Fig. 4 and Supplementary Data 5 ). We tested if the association of the PRS with AD is independent of clinically important factors that are considered in the selection of individuals for clinical trials. First, we showed that the association of the PRS with clinically diagnosed AD cases is similar to the association with pathologically confirmed AD (OR = 1.30 vs. 1.38, per 1-SD increase in the PRS). In this setting, adding variants below the GWS threshold did not lead to a more significant association of the PRS with AD (Fig. 4a ). Next, we tested whether the PRS was associated with AD in the presence of concomitant brain pathologies (besides AD). Among our autopsy-confirmed AD patients ( n = 332), 84% had at least one concomitant pathology, and the PRS was associated with AD in the presence of all tested concomitant pathologies (Fig. 4b ). Moreover, the patients often had more than one concomitant pathology (48.8%), but no difference was observed in the effect estimate of the PRS when more than one pathology was present (Fig. 4b ). Last, we investigated the effect of sex and AAO (Fig. 4c ). 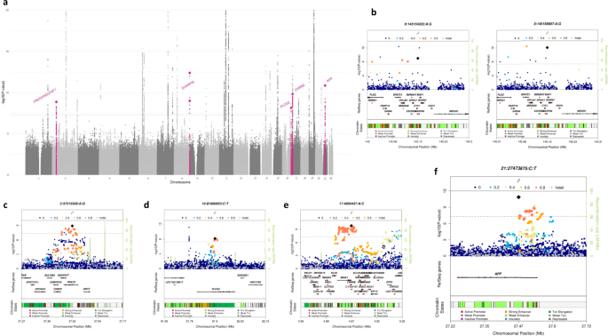Fig. 2: GWAS meta-analysis for AD risk (N= 467,623). aManhattan plot of overall meta-analysis for genome-wide association in Alzheimer’s disease highlighting in pink the loci associated with AD in this study (PRKD3/NDUFAF7, SHARPIN, CHRNE, PLCG2, andAPP).b–fLocus plots for the signals associated with AD in overall meta-analysis results. Our analysis revealed that the effect of the PRS was the same in both sexes (Fig. 4c ) and was consistent with both early-onset (onset before 65 years; OR = 1.58, 95% CI [1.22–2.05], p = 5.8 × 10 −4 ) as well as with late-onset AD (onset later than 85 years; OR = 1.29, 95% CI [1.10–1.51], p = 1.5 × 10 −3 ). Fig. 3: Genetic landscape for Alzheimer’s disease. This figure shows the history of genetic discoveries in AD research over the past 30 years. This figure was constructed to our best knowledge of literature, but is not a systematic review of literature. For common variants, we selected only signals firmly replicated in large meta-GWAS (Lambert et al. [3] , Kunkle et al. [20] , Jun et al. [43] , Sims et al. [7] , Jansen et al. [38] and present study). For rare variants, we only selected those variants widely replicated excluding those loci presenting conflicting results. Abbreviations and more information about the genes can be found in Supplementary Data 4 . The risk alleles associated with AD were represented in orange and the protective alleles in blue. GWAS Genome-Wide Association Study, OR odds ratio. Full size image Fig. 4: Polygenic risk scores for AD. a The 39-SNP PRS association with clinical (OR = 1.30, 95% CI [1.18–1.44], p = 1.1 × 10 −7 ) and pathologically confirmed AD cases (OR = 1.38, per 1-SD increase in the PRS, 95% CI [1.21–1.58], p = 1.5 × 10 −6 ) from EADB–F.ACE/BBB dataset. b PRS association with AD in the presence of concomitant brain pathologies (besides AD). c PRS association with AD stratified by sex and AAO. A similar association of the PRS with AD was found in both sexes (OR males = 1.33, [1.13–1.56], p = 5.8 × 10 −4 vs. OR females = 1.32, [1.19–1.47], p = 2.5 × 10 −7 ). In ( a – c ) data are presented as Odds Ratio per 1-SD increase in PRS (95% CI). The generated PRS was validated using logistic regression adjusted by four principal components. Full size image PRSs has the potential to early identify subjects at risk of complex diseases [24] . To identify people at the highest genetic risk of AD based on the PRS, we used the validated 39-variants PRS in the large GR@ACE dataset. The PRS was associated with a 1.27-fold (95% CI [1.23–1.32]) increased risk for every standard deviation increase in the PRS ( p = 7.3 × 10 −39 ) and with a gradual risk increase when we stratified the dataset into 2% percentiles of the PRS (Fig. 5a , Supplementary Data 6 ). Next, we stratified the dataset in APOE genotype risk groups. The PRS percentiles were associated with AD within the APOE genotype groups (Fig. 5b , Supplementary Data 7 ). Finally, we compared the risk extremes and found a 16.2-fold (95% CI [8.84–29.5], p = 1.5 × 10 −19 ) increased risk for the highest-PRS group ( APOE ɛ4ɛ4 ) compared with the lowest-PRS group ( APOE ɛ2ɛ2/ɛ2ɛ3 ; Supplementary Data 8 ). When we compared the median AAO in AD patients in these extreme risk groups we found a 9-year difference in the median age ( p Wilcoxon = 1.7 × 10 −6 ) (Fig. 5c ). Lastly, we studied the effects on AAO of the PRS in the APOE genotype groups. The PRS differentiated AAO only within APOE ɛ4 carriers. In APOE ɛ4 heterozygotes the PRS determined a 4-year difference in median AAO and in APOE ɛ4 homozygotes ( p Wilcoxon = 6.9 × 10 −5 ), where the PRS determined a median AAO difference of 5.5 years ( p Wilcoxon = 4.6 × 10 −5 ). For the selection of high-risk individuals, it is important to note that we found no difference in the odds and AAO for AD for APOE ɛ4 heterozygotes with the highest PRS compared to APOE ɛ4 homozygotes with the lowest PRS. The Cox regression also showed an impact of APOE on AAO, mainly on APOE ε4ε4 (significant APOE -PRS interaction ( p = 0.021), Fig. 5d , Supplementary Data 9 ). Fig. 5: Polygenic Risk Scores APOE stratification for AD in n = 12,386 biologically independent samples from GR@ACE/DEGESCO. a The AD risk of PRS groups compared to those with the 2% lowest risk. The 2% highest risk had a 3.0-fold (95% CI [2.12–4.18], p = 3.2 × 10 −10 ) increased risk compared with those with the 2% lowest risk. No interaction was found between the PRS and APOE genotypes ( p value = 0.76). b The AD risk stratified by PRS and APOE risk groups compared to the lowest risk group (OR 95% CI). Association was found between highest and lowest-PRS percentiles within the APOE genotype groups: ɛ2ɛ2/ɛ2ɛ3 carriers (OR = 2.48 [1.51–4.08], p = 3.4 × 10 −4 ), ɛ3ɛ3 carriers (OR = 2.67 [1.93–3.69], p = 3.5 × 10 −9 ), ɛ2ɛ4/ɛ3ɛ4 carriers (OR = 2.47 [1.67–3.66], p = 6.8 × 10 −6 ), and ɛ4ɛ4 carriers (OR = 2.02 [1.05–3.85], p = 3.4 × 10 −2 ). Comparisons of the highest and lowest-PRS percentiles with respect to the APOE genotype groups: a difference was found between highest ɛ2ɛ2/ɛ2ɛ3 carriers vs. lowest ɛ3ɛ3 carriers (OR = 0.51 [0.34–0.75], p = 7.8 × 10 −4 ), but not between highest ɛ3ɛ3 carriers vs. lowest ɛ2ɛ4/ɛ3ɛ4 carriers (OR = 1.17 [0.82–1.66], p = 0.40) and highest ɛ2ɛ4/ɛ3ɛ4 carriers vs. lowest ɛ4ɛ4 carriers (OR = 0.89 [0.52–1.53], p = 0.68). c The AAO of AD stratified by PRS and APOE risk groups. No difference in odds for AD was found between the PRS percentiles with AAO in APOE ɛ2ɛ2/ɛ2ɛ3 (lowest = 82 years, highest = 83 years, p Wilcoxon = 0.39) and APOE ɛ3ɛ3 (lowest = 82 years, highest = 81 years, p = 0.16). However, a 4-year difference was found between APOE ɛ4 heterozygotes ( p Wilcoxon = 6.9 × 10 −5 , 81 years compared with 77 years) and 5.5 years difference ( p Wilcoxon = 4.6 × 10 −5 , 78.5 years compared with 73 years) in APOE ɛ4 homozygotes. Data are represented as boxplots as described in the manual of ggplot2 package in R. a – c Logistic regression models adjusted for four population ancestry components were used as statistical test. d Cox regression model on AAO. The determinants are the PRS and the APOE categories, a PRS* APOE interaction term and population substructure as covariates. The curve shows the probability a case in one of the eight groups has developed AD by a certain age ( x -axis). Full size image This work adds on the ongoing global effort to identify genetic variants associated with AD (Fig. 3 ). In the present work, we reported on the largest GWAS for AD risk to date, comprising genetic information of 467,623 individuals of European ancestry. We identified six variants that were not previously associated with the risk of AD and constructed a robust PRS for AD demonstrating its potential value for selecting subjects at risk of AD, especially within APOE ɛ4 carriers. This PRS was based on European ancestries and may or may not generalize to other ancestries. Validation in other populations will be required. We also acknowledge that controls included in GR@ACE are younger than cases and some of the controls might still develop AD later in life. This fact does not invalidate the analysis although reported estimates must be considered conservative. The differences in risk and AAO determined by the PRS of AD are relevant for design clinical trials that over-represent APOE ε4 carriers, as APOE ε4 heterozygous with highest-PRS values have a similar risk and AAO to APOE ɛ4 homozygotes (Fig. 5b ). These represents ~1% of our control population, which is the same percentage as all APOE ε4 homozygotes. A trial that aims to include APOE ɛ4 homozygotes, could consider widening the selection criteria and in this way hasten the enrollment process. Also, our PRS could aid at the interpretation of the results of clinical trials, as it determines a relevant proportion of the AAO, which could either mimic or obscure a treatment effect. The most interesting finding from our GWAS is the discovery of a common protective (MAF (C-allele) = 0.483) intronic variant in the APP gene. Our results directly support APP production or processing as a causal pathway not only in familial AD but in common sporadic AD. The SNP is in a DNase hypersensitive area of 295 bp (chr21:27473781-27474075) possibly involved in the transcriptional regulation of the APP gene. rs2154481 is an eQTL for the APP mRNA and an antisense transcript of the APP gene named AP001439.2 in public eQTL databases [25] (Supplementary Fig. 4 ). Functional evidence supports a modified APP transcription [26] as an LD block of 13 SNPs within the APP locus (including rs2154481) increased the TFCP2 transcription factor avidity to its binding site and increased the enhancer activity of this specific intronic region [26] . Based on this evidence, we can postulate that a life-long slightly higher APP gene expression protects the brain from AD insults. Still, this seems counterintuitive as duplications of the gene lead to early-onset AD [27] . A U-shaped effect, or hormesis effect of APP might help explain our observations and it might also fit the accelerated cognitive deterioration observed in AD patients treated with beta-secretase inhibitors [28] , [29] as these reduce beta-amyloid in their brain. An alternative hypothesis is that mechanisms underlying the variant are related to the overexpression of protective fragments of the APP protein [30] . Disentangling the molecular mechanism of our finding will help refine and steer the amyloid hypothesis. Additionally, other three variants identified are altering protein sequence or affecting regulatory motifs. Two independent missense mutations in SHARPIN increased the AD risk. SHARPIN was previously proposed as an AD candidate gene [31] , [32] , and functional analysis of a rare missense variant (NM_030974.3:p.Gly186Arg) resulted in the aberrant cellular localization of the variant protein and attenuated the activation of NF-κB, a central mediator of inflammatory and immune responses. Functional analysis of the two identified missense variants will show if the effect on immune reaction in AD is similar. The variant located in the CHRNE which encodes a subunit of the cholinergic receptor (AChR) is a strong modulator of CHRNE expression. The same allele that increases AD risk increases the expression in the brain and other tissues according to GTEx ( p = 2.1 × 10 −13 ) (Supplementary Fig. 5 ). The detection of a potential hypermorph allele linked to AD risk and affecting cholinergic function could reintroduce this neurotransmitter pathway into the search for preventative strategies. Further functional studies are needed to consolidate this hypothesis. Altogether, we described six additional loci associated with sporadic AD. These signals reinforce that AD is a complex disease in which amyloid processing and immune response play key roles. We add to the growing body of evidence that the polygenic scores of all genetic loci to date, in combination with APOE genotypes, are robust tools that are associated with AD and its AAO. These properties make PRS promising in selecting individuals at risk to apply preventative therapeutic strategies. Data Participants in this study were obtained from multiple sources, including raw data from case-control samples collected by GR@ACE/DEGESCO, summary statistics data from the case-control samples in the IGAP and the summary statistics of AD-by-proxy phenotype from the UK Biobank. An additional case-control samples from 16 independent cohorts (19,087 AD cases and 39,101 controls) was used for replication, largely collected and analyzed by the European Alzheimer’s Disease Biobank (JPND-EADB) project. Full descriptions of the samples and their respective phenotyping and genotyping procedures are provided in the Supplementary Methods . GR@ACE The GR@ACE study [19] recruited AD patients from Fundació ACE, Institut Català de Neurociències Aplicades (Catalonia, Spain), and control individuals from three centers: Fundació ACE (Barcelona, Spain), Valme University Hospital (Seville, Spain), and the Spanish National DNA Bank–Carlos III (University of Salamanca, Spain) ( http://www.bancoadn.org ). Additional cases and controls were obtained from dementia cohorts included in the Dementia Genetics Spanish Consortium (DEGESCO) [33] . At all sites, AD diagnosis was established by a multidisciplinary working group—including neurologists, neuropsychologists, and social workers—according to the DSM-IV criteria for dementia and the National Institute on Aging and Alzheimer’s Association’s (NIA–AA) 2011 guidelines for diagnosing AD. In our study, we considered as AD cases any individuals with dementia diagnosed with probable or possible AD at any point in their clinical course. For further details on the contribution of the sites, see Supplementary Data 10 . Written informed consent was obtained from all the participants. The ethics and scientific committees have approved this research protocol (Acta 25/2016, Ethics Committee H., Clinic I Provincial, Barcelona, Spain). Genotyping, quality control, and imputation . DNA was extracted from peripheral blood according to standard procedures using the Chemagic system (Perkin Elmer). Samples reaching DNA concentrations of >10 ng/µl and presenting high integrity were included for genotyping. Cases and controls were randomized across sample plates to avoid batch effects. Genotyping was conducted using the Axiom 815K Spanish biobank array (Thermo Fisher) at the Spanish National Center for Genotyping (CeGEN, Santiago de Compostela, Spain). The genotyping array not only is an adaptation of the Axiom biobank genotyping array but also contains rare population-specific variations observed in the Spanish population. The DNA samples were genotyped according to the manufacturer’s instructions (Axiom™ 2.0 Assay Manual Workflow). The Axiom 2.0 assay interrogates biallelic SNPs and simple indels in a single-assay workflow. Starting with 200 ng of genomic DNA, the samples were processed through a manual target preparation protocol, followed by automated processing of the array plates in the GeneTitan Multi-Channel (MC) instrument. Target preparation involved DNA amplification, fragmentation, purification, and resuspension of the target in a hybridization cocktail. The hyb-ready targets were then transferred to the GeneTitan MC instrument for automated, hands-free processing, including hybridization, staining, washing, and imaging. The CEL files were generated using the GeneTitan MC instrument. Quality control (QC) was performed for samples and plates using the Affymetrix power tool (APT) 1.15.0 software following the Axiom data analysis workflow. The sample quality was determined based on the resolution of AT and GC channels in a group of non-polymorphic SNPs (resolution > 0.82). Samples with a call rate greater than 97% and plates with an average call rate above 98.5% were included for final SNP calling. The samples were jointly called. Markers passing all the QC tests were used in downstream analysis ( N SNPs = 729,868; 95.4%) using the SNPolisher R package (Thermo Fisher). To assess the sample genotyping concordance, we intentionally resampled 200 samples and determined a concordance rate of 99.5%. We also conducted previously described standard QC prior to imputation [19] . In brief, individual QC includes genotype call rates >97%, sex checks, and no excess heterozygosity; we removed population outliers as well (European cluster of 1000 Genomes). We included variants with a call rate of >95%, with a minor allele frequency (MAF) of >0.01, in Hardy–Weinberg equilibrium ( p < 1 × 10 −4 in controls) and without differential missingness between cases and controls (Supplementary Data 11 , Supplementary Fig. 1 ). Imputation was carried out using the Haplotype reference consortium [34] (HRC, full panel) and the 1000 Genomes reference panel [35] (for indels only) on the Michigan Imputation Server ( https://imputationserver.sph.umich.edu ). Rare variants (MAF < 0.001) and variants with low imputation quality ( R 2 < 0.30) were excluded. Logistic regression models, adjusted for the first four ancestry principal components [19] , were fitted using Plink (v2.00a). Population-based controls were used; therefore, age was not included as a covariate. Age and gender statistically behave like phenotype proxies (for AD status in this case). Therefore, adjusting for co-variation with age and gender could result in an over-adjustment of GWAS results. After QC steps, we included 6,331 AD cases and 6,055 control individuals and tested 14,542,816 genetic variants for association with AD. IGAP summary statistics The GWAS summary results from the IGAP were downloaded from the National Institute on Aging Genetics of Alzheimer’s Disease Data Storage Site (NIAGADS, https://www.niagads.org/ ) [20] . Details on data generation and analyses by the IGAP have been previously described [20] . In brief, the IGAP is a large study based upon genome-wide association using individuals of European ancestry. Stage 1 of the IGAP comprises 21,982 AD cases and 41,944 cognitively normal controls from four consortia: the Alzheimer Disease Genetics Consortium (ADGC), the European Alzheimer’s Disease Initiative (EADI), the Cohorts for Heart and Aging Research in Genomic Epidemiology (CHARGE) Consortium, and the Genetic and Environmental Risk in AD/Defining Genetic, Polygenic, and Environmental Risk for Alzheimer’s Disease (GERAD/PERADES) Consortium. Summary statistics are available for 11,480,632 variants, both genotyped and imputed (1000 Genomes phase 1, v3). In Stage 2, 11,632 SNPs were genotyped in an independent set of 8362 AD cases and 10,483 controls. 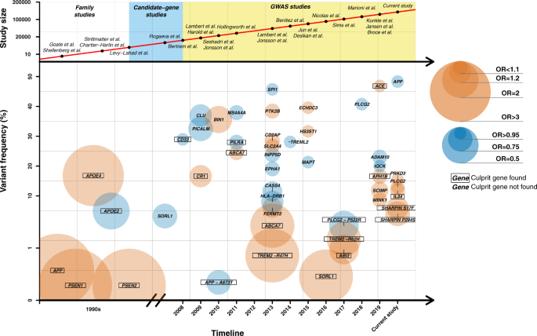Fig. 3: Genetic landscape for Alzheimer’s disease. This figure shows the history of genetic discoveries in AD research over the past 30 years. This figure was constructed to our best knowledge of literature, but is not a systematic review of literature. For common variants, we selected only signals firmly replicated in large meta-GWAS (Lambert et al.3, Kunkle et al.20, Jun et al.43, Sims et al.7, Jansen et al.38and present study). For rare variants, we only selected those variants widely replicated excluding those loci presenting conflicting results. Abbreviations and more information about the genes can be found in Supplementary Data4. The risk alleles associated with AD were represented in orange and the protective alleles in blue. GWAS Genome-Wide Association Study, OR odds ratio. UK Biobank summary statistics UK Biobank data—including health, cognitive, and genetic data—was collected on over 500000 individuals aged 37–73 years from across Great Britain (England, Wales, and Scotland) at the study baseline (2006–2010) ( http://www.ukbiobank.ac.uk ) [36] . Several groups have demonstrated the utility of self-report of parental history of AD for case ascertainment in GWAS (proxy–AD approach) [21] , [37] , [38] . For this study, we used the published summary statistics of Marioni et al. [21] . They included, after stringent QC, 314,278 unrelated individuals for whom AD information was available on at least one parent in the UK Biobank ( https://datashare.is.ed.ac.uk/handle/10283/3364 ). In brief, the 27,696 participants whose mothers had dementia (maternal cases) were compared with the 260,980 participants whose mothers did not have dementia. Likewise, the 14,338 participants whose fathers had dementia (paternal cases) were compared with the 245,941 participants whose fathers did not have dementia [21] . The phenotype of the parents is independent, and therefore, the estimates could be meta-analyzed. After analysis, the effect estimates were made comparable to a case-control setting. Further information on the transformation of the effect sizes can be found elsewhere [21] , [39] . The data available comprises summary statistics of 7,794,553 SNPs imputed to the HRC reference panel (full panel). Meta-GWAS of AD After study-specific variant filtering and quality-control procedures, we performed a fixed effects inverse-variance–weighted meta-analysis [22] on the discovery and follow-up stages (Supplementary Data 1 and Supplementary Data 12 ). To determine the lead SNPs (those with the strongest association per genomic region), we performed clumping on SNPs with a GWS p value ( p < 5 × 10 −8 ) (Plink v1.90, maximal linkage disequilibrium (LD) with R 2 < 0.001 and physical distance 250 Kb). In the APOE region, we only considered the APOE ɛ4 (rs429358) and APOE ɛ2 (rs7412) SNPs [40] . LD information was calculated using the GR@ACE imputed genotypes as a reference. Polygenicity and confounding biases, such as cryptic relatedness and population stratification, can yield an inflated distribution of test statistics in GWAS. To distinguish between inflation from a true polygenic signal and bias we quantified the contribution of each by examining the relationship between test statistics and linkage disequilibrium (LD) using the LD Score regression intercept (LDSC software [41] ). Chromosomal regions associated with AD in previous studies were excluded from follow-up (Lambert et al. [3] , Kunkle et al. 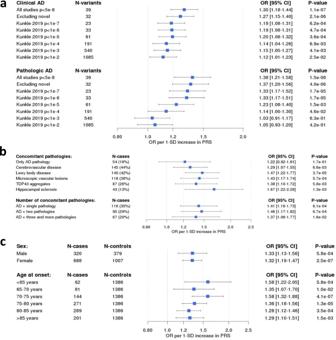Fig. 4: Polygenic risk scores for AD. aThe 39-SNP PRS association with clinical (OR = 1.30, 95% CI [1.18–1.44],p= 1.1 × 10−7) and pathologically confirmed AD cases (OR = 1.38, per 1-SD increase in the PRS, 95% CI [1.21–1.58],p= 1.5 × 10−6) from EADB–F.ACE/BBB dataset.bPRS association with AD in the presence of concomitant brain pathologies (besides AD).cPRS association with AD stratified by sex and AAO. A similar association of the PRS with AD was found in both sexes (ORmales= 1.33, [1.13–1.56],p= 5.8 × 10−4vs. ORfemales= 1.32, [1.19–1.47],p= 2.5 × 10−7). In (a–c) data are presented as Odds Ratio per 1-SD increase in PRS (95% CI). The generated PRS was validated using logistic regression adjusted by four principal components. 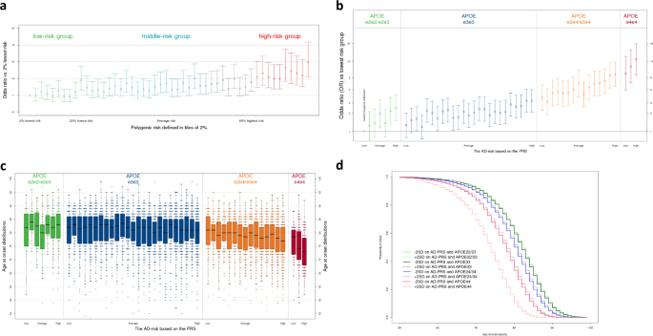Fig. 5: Polygenic Risk ScoresAPOEstratification for AD inn= 12,386 biologically independent samples from GR@ACE/DEGESCO. aThe AD risk of PRS groups compared to those with the 2% lowest risk. The 2% highest risk had a 3.0-fold (95% CI [2.12–4.18],p= 3.2 × 10−10) increased risk compared with those with the 2% lowest risk. No interaction was found between the PRS andAPOEgenotypes (pvalue = 0.76).bThe AD risk stratified by PRS andAPOErisk groups compared to the lowest risk group (OR 95% CI). Association was found between highest and lowest-PRS percentiles within theAPOEgenotype groups:ɛ2ɛ2/ɛ2ɛ3carriers (OR = 2.48 [1.51–4.08],p= 3.4 × 10−4),ɛ3ɛ3carriers (OR = 2.67 [1.93–3.69],p= 3.5 × 10−9),ɛ2ɛ4/ɛ3ɛ4carriers (OR = 2.47 [1.67–3.66],p= 6.8 × 10−6), andɛ4ɛ4carriers (OR = 2.02 [1.05–3.85],p= 3.4 × 10−2). Comparisons of the highest and lowest-PRS percentiles with respect to theAPOEgenotype groups: a difference was found between highestɛ2ɛ2/ɛ2ɛ3carriers vs. lowestɛ3ɛ3carriers (OR = 0.51 [0.34–0.75],p= 7.8 × 10−4), but not between highestɛ3ɛ3carriers vs. lowestɛ2ɛ4/ɛ3ɛ4carriers (OR = 1.17 [0.82–1.66],p= 0.40) and highestɛ2ɛ4/ɛ3ɛ4carriers vs. lowestɛ4ɛ4carriers (OR = 0.89 [0.52–1.53],p= 0.68).cThe AAO of AD stratified by PRS andAPOErisk groups. No difference in odds for AD was found between the PRS percentiles with AAO inAPOE ɛ2ɛ2/ɛ2ɛ3(lowest = 82 years, highest = 83 years,pWilcoxon= 0.39) andAPOE ɛ3ɛ3(lowest = 82 years, highest = 81 years,p= 0.16). However, a 4-year difference was found betweenAPOE ɛ4heterozygotes (pWilcoxon= 6.9 × 10−5, 81 years compared with 77 years) and 5.5 years difference (pWilcoxon= 4.6 × 10−5, 78.5 years compared with 73 years) inAPOE ɛ4homozygotes. Data are represented as boxplots as described in the manual of ggplot2 package in R.a–cLogistic regression models adjusted for four population ancestry components were used as statistical test.dCox regression model on AAO. The determinants are the PRS and theAPOEcategories, a PRS*APOEinteraction term and population substructure as covariates. The curve shows the probability a case in one of the eight groups has developed AD by a certain age (x-axis). [42] , and Jansen et al. [38] ). We tested all variants with suggestive association ( p < 10 −5 ) located in proximity (200 kb) of genomic regions selected for follow-up to allow for the potential refinement of the top associated variant. Conditional analyses were performed in regions where multiple variants were associated with AD using logistic regression models, adjusting for the genetic variants in the region (Supplementary Data 13 , 14 ). Regional plots were generated with a mixture of homemade Python (v2.7) and R (v3.6.0) scripts. Briefly, given an input variant, we calculated the LD between the input variant and all the surrounding variants within a window of length defined by the user. The LD was calculated in the 1000 Genomes samples of European ancestry. We used gene positions from RefSeq (release 93); in the case of multiple gene models for a given gene, we reported the model with the largest number of exons. We used recombination rates from HapMap II and chromatin states from ENCODE/Broad (15 states were grouped to highlight the predicted functional elements). As a reference genome, we used GRCh37. Quantile–quantile plots, Manhattan plots, and the exploration of genomic inflation factors were performed using the R package qqman. Polygenic risk scores We calculated a weighted individual PRS based on the 39 genetic variants that showed GWS evidence of association with AD in the present study, excluding APOE to check the impact of PRS modulating APOE risk (Table 1 and Supplementary Data 3 ). The selected variants were directly genotyped or imputed with high quality (median imputation score R ² = 0.93). The PRSs were generated by multiplying the genotype dosage of each risk allele for each variant by its respective weight and then summing across all variants. We weighted this by the effect size from previous IGAP studies [Kunkle et al. [42] (36 variants), Sims et al. [7] (2 variants), Jun et al. [43] ( MAPT locus), Supplementary Data 5 ]. The generated PRS was validated using logistic regression adjusted by four principal components in a sample of 676 AD cases diagnosed based on clinical criteria and 332 pathologically confirmed AD cases from the European Alzheimer’s Disease Biobank–Fundació ACE/Barcelona Brain Bank dataset (EADB–F.ACE/BBB, Supplementary Information ). This dataset was not used in prior genetic studies. In this dataset, all pathologically confirmed cases were scored for the presence or absence of concomitant pathologies. In all analyses, we compared the AD patients to the same control dataset ( n = 1386). We performed analyses to test the robustness of the PRS. We tested the effect of adding variants below the genome-wide significance threshold using a pruning and thresholding approach. For this, we used the summary statistics of the IGAP [42] study, and we selected independent variants using the clump_data() function from the TwoSampleMR package (v0.4.25). We used strict settings for clumping ( R 2 = 0.001 and window = 1 MB) and increasing p value thresholds (>1 × 10 −7 , >1 × 10 −6 , >1 × 10 −5 , >1 × 10 −4 , >1 × 10 −3 , and >1 × 10 −2 ). We tested the association of the results with clinically diagnosed and pathologically confirmed AD patients. To evaluate the effect of diagnostic certainty, we tested whether the PRS was different between the two patient groups. For the PRS with 39 GWS variants, we tested whether the PRS had sex-specific effects, whether it resulted in different age-of-onset groups of AD, and the effect of the PRS in the presence of concomitant brain pathologies. Risk stratification of the validated PRSs . We searched for the groups at the highest risk of AD in the GR@ACE dataset (6331 AD cases and 6055 controls). We stratified the population into PRS percentiles, taking into account survival bias anticipated at old age [18] . To eliminate selection bias, we calculated the boundaries of the percentiles in the control participants aged 55 years and younger ( n = 3546). Based on the boundaries from this population, the rest of the controls and all AD cases were then assigned into their appropriate percentiles. We first explored risk stratification using only the PRSs. For this, we split the PRSs into 50 groups (2 percentiles) and compared all groups with that which had the lowest PRS. Second, we explored risk stratification considering both the APOE genotypes and the PRSs. The APOE genotypes were pooled in the analyses as APOE ɛ2ɛ2/ɛ2ɛ3 ( n = 998, split into 7 PRS groups), APOE ɛ3ɛ3 ( n = 7611, split into 25 PRS groups), APOE ɛ2ɛ4/ɛ3ɛ4 ( n = 3399, split into 15 PRS groups), and APOE ɛ4ɛ4 ( n = 382, split into 3 PRS groups). We studied the effect of PRS across groups of individuals stratified by the APOE genotypes with the lowest-PRS group ( APOE as the reference group using logistic regression models adjusted for four population ancestry components). Finally, we compared the median AAO using a Wilcoxon test. We implemented a Cox regression model on AAO in the GR@ACE/DEGESCO dataset case-only adjusted for covariates as APOE group, the interaction between the PRS and APOE and four population ancestry components. All analyses were done in R (v3.4.2). Functional annotation We used Functional Mapping and Annotation of Genome-Wide Association Studies [23] (FUMA, v1.3.4c) to interpret SNP-trait associations (see Supplementary Methods and Supplementary Data 15 – 18 ). FUMA is an online platform that annotates GWAS findings and prioritizes the most likely causal SNPs and genes using information from 18 biological data repositories and tools. As input, we used the summary statistics of our meta-GWAS. Gene prioritization is based on a combination of positional mapping, expression quantitative trait loci (eQTL) mapping, and chromatin interaction mapping. Functional annotation was performed by applying a methodology similar to that described by Jansen et al. [38] . We referred to the original publication for details on the methods and repositories of FUMA [23] . Reporting summary Further information on research design is available in the Nature Research Reporting Summary linked to this article.